Large-scale analysis of lysine SUMOylation by SUMO remnant immunoaffinity profiling Small ubiquitin-related modifiers (SUMO) are evolutionarily conserved ubiquitin-like proteins that regulate several cellular processes including cell cycle progression, intracellular trafficking, protein degradation and apoptosis. Despite the importance of protein SUMOylation in different biological pathways, the global identification of acceptor sites in complex cell extracts remains a challenge. Here we generate a monoclonal antibody that enriches for peptides containing SUMO remnant chains following tryptic digestion. We identify 954 SUMO3-modified lysine residues on 538 proteins and profile by quantitative proteomics the dynamic changes of protein SUMOylation following proteasome inhibition. More than 86% of these SUMOylation sites have not been reported previously, including 5 sites on the tumour suppressor parafibromin (CDC73). The modification of CDC73 at K136 affects its nuclear retention within PML nuclear bodies on proteasome inhibition. In contrast, a CDC73 K136R mutant translocates to the cytoplasm under the same conditions, further demonstrating the effectiveness of our method to characterize the dynamics of lysine SUMOylation. The small ubiquitin-related modifier (SUMO) is a ubiquitin-like (UBL) protein that is reversibly conjugated to a wide range of substrates involved in different regulatory pathways including intracellular trafficking, cell cycle, genome integrity, protein degradation, cell differentiation and apoptosis [1] , [2] , [3] , [4] , [5] , [6] . Protein SUMOylation is carried out by an enzymatic cascade consisting of the E1 SUMO-activating enzyme (SAE1/SAE2), E2 SUMO-conjugating enzyme (Ubc9) and one of several E3 SUMO ligases [4] , [5] . DeSUMOylation is performed by Sentrin/SUMO-specific proteases, a family of conserved proteins that can also process SUMO precursors to expose the carboxy-terminal diglycine motif of mature SUMO proteins for its conjugation to the side chains of lysine residues in target proteins [7] . Although protein SUMOylation is commonly observed on lysine residues of the canonical consensus sequence ψK x E (where ψ is a hydrophobic residue and x any amino acid) recognized by Ubc9, SUMO-acceptor sites cannot be predicted accurately as many proteins with this motif are not SUMOylated and this modification is also found at non-consensus sites [8] . As for other UBLs, SUMOylation can occur at distinct sites on the same protein substrate and can undergo self-modification to form polySUMO chains that mediate the recruitment of effector proteins containing SUMO-interacting motifs [9] , [10] . Detailed understanding of the functional and physiological significance of protein SUMOylation requires specific enrichment approaches enabling the large-scale detection of SUMO targets from complex cell extracts. This is necessary in view of the highly dynamic nature of this modification and the relatively low abundance of SUMOylated proteins. Consequently, large efforts have been deployed over the past decade to develop protocols and tools to facilitate their analysis. Our group and others have used His-tagged SUMO to enrich potential targets using immobilized metal affinity chromatography (IMAC) under denaturing conditions [11] , [12] , [13] . Affinity purification using IMAC and/or immunoprecipitation have been successfully applied to the large-scale analysis of SUMOylated proteins from different model organisms, including Saccharomyces cerevisiae [14] , [15] , [16] , Drosophila melanogaster [17] , Arabidopsis thaliana [18] and mammalian cells [11] , [12] , [19] , [20] , [21] . The combination of these affinity approaches with quantitative proteomics using label-free or metabolic labelling have also expanded the repertoire of protein substrates regulated by heat shock or stress conditions [18] , [19] , [22] , [23] , [24] . Global or individual detection of endogenous SUMOylated substrates has been notoriously more challenging and was reported only in a limited number of cases. For example, Bruderer et al. [25] have exploited the presence of 4 SUMO-interacting motif domains on the poly-SUMO-dependent ubiquitin E3 ligase RNF4 to identify more than 300 poly-SUMOylated proteins in HeLa cells following heat-shock treatment. A recent report described the use of commercial monoclonal antibodies to SUMO1 and SUMO2/3 for the analysis of individual SUMOylated proteins and global SUMO proteome analyses of mammalian cells and tissues [26] . Although these protocols are effective to purify and quantify SUMOylated proteins from different cell model systems, the precise identification of modified residues by mass spectrometry (MS) is significantly more difficult, and has been reported only in a few instances. This is due in part to the low stoichiometry of protein SUMOylation and the relatively long SUMO remnant appended on lysine residues following tryptic digestion (for example, up to 32 amino acids for SUMO2/3). The branched structure of the corresponding peptides not only complicates the interpretation of the MS/MS spectra, but often require specialized pattern recognition tools or database search engines such as SUMmOn [27] or ChopNSpice [28] to facilitate their identification. Here we developed a novel proteomics approach for antibody-based capture and MS analyses of SUMO-modified peptides. We took advantage of HEK293 cell lines stably expressing SUMO mutants [11] to generate a monoclonal antibody that specifically recognize SUMO remnants left after tryptic digestion of SUMOylated proteins. We demonstrated the feasibility of this approach using HEK293 cells expressing a modified form of SUMO3 and identified 954 unique SUMOylation sites on 538 SUMOylated protein substrates. More than 86% of the identified sites were previously unknown, including five SUMOylation sites on the tumour suppressor parafibromin (cell division cycle 73, CDC73) that were regulated by proteasome inhibition. Site-directed mutagenesis and immunofluorescence experiments indicated that SUMOylation of CDC73 K136 affects its nucleocytoplasmic localization. These results demonstrate the effectiveness of our approach to characterize the global dynamics of lysine SUMOylation and to investigate the functional significance of this modification in different cellular processes. Immunoaffinity enrichment of SUMO remnant peptides In the present study, we used HEK293 cell lines stably expressing SUMO (1, 2 or 3) mutant proteins that contain an amino-terminal His 6 tag and a strategically located arginine residue near the C terminus, similar to that found in the yeast Smt3 protein ( Fig. 1a ) [11] . We hereafter refer to these proteins as SUMOm to indicate the presence of the N-terminal His 6 tag and the insertion of an arginine near the C terminus. On tryptic digestion, protein targets conjugated with these altered forms of SUMO generate short SUMO remnants on modified lysine residues that are unique to each paralogue and facilitate the identification of SUMOylation sites. The activity and functional properties of our three forms of SUMOm are similar to those of wild-type (WT) SUMO proteins and were validated by in vitro SUMOylation assays and immunofluorescence microscopy experiments [11] . To identify SUMOylated proteins and their corresponding sites of modification, we generated a monoclonal antibody that recognizes peptides containing the SUMO remnant left after trypsin digestion. This was achieved by conjugating peptides F{(EQTGG)K}GEC and F{(NQTGG)K}GEC to the keyhole limpet haemocyanin protein via the cysteine residue (Methods). We injected the corresponding immunogens into rabbits and screened hybridoma lines for antibodies that specifically recognize peptides with the SUMO remnant on modified lysine residues. Hybridoma line UMO 1-7-7 produced a monoclonal antibody that showed higher specificity towards the EQTGG and NQTGG epitopes. To determine whether the UMO 1-7-7 antibody was able to immunoprecipitate peptides containing the SUMO remnant from each paralogue, we spiked six different synthetic peptides at concentration of 20 and 50 nM in a tryptic digest of HEK293 cells not expressing SUMO mutants. Immunoprecipitation of the corresponding tryptic digest with this antibody resulted in a selective enrichment of peptides containing the SUMO remnant lysine ( Supplementary Fig. 1a ). We evaluated the quantitative recovery of SUMO peptides following immunoaffinity enrichment and obtained more than 50% yield on average ( Supplementary Fig. 1b ). To determine the diversity of peptide sequences that can be recognized by the UMO 1-7-7 antibody, we also spiked 66 synthetic peptides containing a SUMO3m remnant chain at a concentration level of 50 nM into a tryptic digest of proteins from HEK293 cells. Liquid chromatography-tandem MS (LC-MS/MS) analysis of this sample enabled the identification of 3,092 peptides including all synthetic peptides. In contrast, the LC-MS/MS analysis of the immunoaffinity-enriched sample identified 121 peptides, of which 60 corresponded to our synthetic peptides with SUMO3m remnants ( Supplementary Fig. 2 ). These experiments demonstrated that the UMO 1-7-7 antibody is capable of enriching peptides containing SUMO remnant-modified lysines with high specificity. 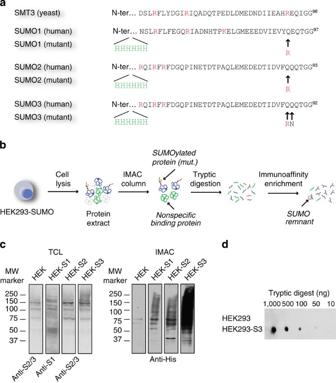Figure 1: SUMO remnant immunoaffinity purification strategy. (a) The sequence of SMT3 (S. cerevisiae) and three human SUMO paralogues. Mutant SUMO (SUMOm) proteins were produced each containing a His6at the N terminus and an Arg residue at the sixth position from the C terminus. The Q88N mutation was inserted in SUMO3 so that it can be distinguished from the SUMO2 mutant paralogue. (b) Overview of the SUMOm remnant immunoaffinity purification. Cell lysates were separated on an IMAC column to enrich SUMOylated proteins before tryptic digestion. Tryptic peptides containing the five amino acid SUMOm remnant were enriched using the UMO 1-7-7 monoclonal antibody. (c) Detection of SUMOylated proteins from nuclear extracts of HEK293-SUMOm cells before and after IMAC purification using anti-His, anti-SUMO1 and anti-SUMO2/3 antibodies. (d) Enriched SUMOylated proteins from HEK293 SUMO3m cells were digested with trypsin and probed for SUMO remnant tryptic peptides using the UMO 1-7-7 monoclonal antibody. Figure 1: SUMO remnant immunoaffinity purification strategy. ( a ) The sequence of SMT3 ( S. cerevisiae ) and three human SUMO paralogues. Mutant SUMO (SUMOm) proteins were produced each containing a His 6 at the N terminus and an Arg residue at the sixth position from the C terminus. The Q88N mutation was inserted in SUMO3 so that it can be distinguished from the SUMO2 mutant paralogue. ( b ) Overview of the SUMOm remnant immunoaffinity purification. Cell lysates were separated on an IMAC column to enrich SUMOylated proteins before tryptic digestion. Tryptic peptides containing the five amino acid SUMOm remnant were enriched using the UMO 1-7-7 monoclonal antibody. ( c ) Detection of SUMOylated proteins from nuclear extracts of HEK293-SUMOm cells before and after IMAC purification using anti-His, anti-SUMO1 and anti-SUMO2/3 antibodies. ( d ) Enriched SUMOylated proteins from HEK293 SUMO3m cells were digested with trypsin and probed for SUMO remnant tryptic peptides using the UMO 1-7-7 monoclonal antibody. Full size image We next sought to determine the efficiency of this antibody to enrich SUMOylated lysines in HEK293 cells expressing each SUMOm paralogue. To reduce sample complexity before tryptic digestion and immunoaffinity purification, we enriched His 6 -tagged SUMOylated proteins using IMAC. A work flow illustrating the sample preparation, IMAC purification, trypsin digestion and immunoprecipitation is shown in Fig. 1b . Enrichment of SUMOylated proteins (SUMO1m, SUMO2m or SUMO3m) was clearly observed on the anti-SUMO immunoblots from nuclear extracts obtained before and after IMAC purification ( Fig. 1c ). In contrast, no enrichment of endogenous SUMOylated proteins was shown in nuclear extracts from control HEK293 cells (that is, cells not expressing SUMOm). Enriched SUMOylated proteins were subsequently digested with trypsin to compare the ability of our monoclonal antibody to recognize SUMOylated peptides containing paralogue-specific SUMO remnants. Dot blots performed on tryptic digests of HEK293 cells expressing SUMO3m showed staining patterns consistent with sample loadings, whereas no signal was detected for digests from control HEK293 cells ( Fig. 1d ). These results indicated that the antibody specifically recognizes SUMOm remnants on modified lysines, and that tryptic peptides from control HEK293 cells not expressing SUMOm showed no significant cross-reactivity. To determine the repertoire of SUMO peptides pulled down by the antibody, we immunoprecipitated peptides from tryptic digests of IMAC-purified nuclear extracts from HEK293 cells stably expressing each SUMOm paralogue and analysed the corresponding samples by online two-dimensional (2D)-LC-MS/MS. A comparison of total ion chromatograms obtained before and after immunoprecipitation of extracts from HEK293 cells expressing SUMO3m is shown in Fig. 2a and highlights the different distribution of peptides for these two samples. The inset of Fig. 2a also shows the extracted ion chromatograms for m/z 732.05 corresponding to the tryptic peptide LEGH K EGIVQTEQIR from parafibromin (CDC73) with a SUMOylated K301 residue. The tumour suppressor CDC73 is a component of the RNA polymerase-associated factor 1 complex [29] and was not previously known to be SUMOylated. The presence of this peptide in the tryptic digest of the IMAC-purified extract was barely detectable in the extracted MS spectrum of the corresponding peak ( Fig. 2b , left panel). However, this peptide showed a 12-fold enrichment on immunoprecipitation ( Fig. 2b , right panel) and was readily identified following a Mascot search ( Fig. 2c ). The higher energy collisional dissociation (HCD) MS/MS spectrum shown in Fig. 2c also revealed structural features consistent with those previously observed for branched SUMO peptides [30] . In particular, we note the presence of fragment ions from the SUMO3m remnant chain ( m/z 132.077 ( c 1 *), 226.082 ( b 2 *-NH 3 ), 243.109 ( b 2 *), 344.157 ( b 3 *), where * indicates fragment on remnant SUMO chain), neutral losses (NQ: 242.101 Da, NQT: 343.249 Da, NQTG: 400.171 Da, NQTGG: 457.192 Da) of the SUMO3m remnant for the multiply protonated precursor ion and y -type fragment ions containing the modified lysine residue. Although fragment ions from the short SUMOm remnant can be advantageously exploited to validate SUMOylated peptides, they give rise to more complex MS/MS spectra than linear peptides, which results in reduced identifications and lower scores using standard database search engines. To maximize SUMOylated peptide identification, we developed a script that use paralogue-specific fragment ion features observed in HCD collisional activation to retrieve MS/MS spectra of SUMOylated peptide candidates and remove the corresponding fragment ions from the MS/MS spectra before Mascot searches ( Supplementary Fig. 3 ). This script is different from that reported recently [30] and takes into account cleavages of residues within the SUMO3m remnant (for example, y 11 -NQ, y 11 -NQT and y 11 -NQTG in Fig. 2c ). A comparison of the search output obtained using Mascot with and without removal of SUMO fragment ions indicated that the removal of SUMO3m fragment ions led to an 11% increase of Mascot scores and provided a 41% gain in new identification of SUMOylation sites compared with conventional searches ( Supplementary Fig. 4 ). 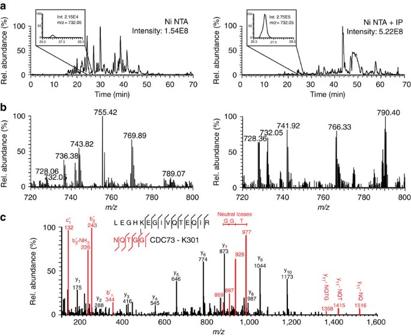Figure 2: Enrichment of SUMOylated peptides using SUMO remnant immunoaffinity purification. (a) LC-MS/MS analyses of tryptic digests from IMAC-purified proteins before and after immunoaffinity purification. Insets show the extracted ion chromatograms for the triply protonated peptide ion of SUMOylated K301 from CDC73 atm/z732.05. The SUMOylated peptide is clearly detected following immunoaffinity with a 12-fold enrichment compared with the IMAC purification alone. (b) Extracted mass spectra of the corresponding SUMOylated peptide from LC-MS/MS analysis of IMAC-purified proteins before (right) and after (left) immunoaffinity purification. (c) MS/MS spectrum of the tryptic peptidem/z732.05 from CDC73 with SUMOylated K301. SUMO remnant fragments ions (m/z132, 226, 243, 344, 869,897, 926, 977) and the neutral losses (−NQ, −NQT, −NQTG, −NQTGG) are highlighted in red and confirmed the sequence assignment. Figure 2: Enrichment of SUMOylated peptides using SUMO remnant immunoaffinity purification. ( a ) LC-MS/MS analyses of tryptic digests from IMAC-purified proteins before and after immunoaffinity purification. Insets show the extracted ion chromatograms for the triply protonated peptide ion of SUMOylated K301 from CDC73 at m/z 732.05. The SUMOylated peptide is clearly detected following immunoaffinity with a 12-fold enrichment compared with the IMAC purification alone. ( b ) Extracted mass spectra of the corresponding SUMOylated peptide from LC-MS/MS analysis of IMAC-purified proteins before (right) and after (left) immunoaffinity purification. ( c ) MS/MS spectrum of the tryptic peptide m/z 732.05 from CDC73 with SUMOylated K301. SUMO remnant fragments ions ( m/z 132, 226, 243, 344, 869,897, 926, 977) and the neutral losses (−NQ, −NQT, −NQTG, −NQTGG) are highlighted in red and confirmed the sequence assignment. Full size image SUMO proteome dynamics following proteasome inhibition We combined this newly developed immunoaffinity purification method with label-free quantitative proteomics, to determine global changes in protein SUMOylation following cell treatment with the proteasome inhibitor MG132 ( Fig. 3a , Methods). Previous reports indicated that significant cross-talk exists between SUMO2/3 and the ubiquitin–proteasome system, and control many target proteins that regulate different aspects of nucleic acid metabolism [31] . We profiled temporal changes in protein SUMOylation in HEK293 cells expressing SUMO3m on proteasome inhibition and obtained maximum SUMOylation for cells treated overnight with 10 μM of MG132 ( Supplementary Fig. 5 ). Nuclear extracts from control and MG132-treated cells were isolated, purified on IMAC column and digested with trypsin. For each sample, enrichment of SUMOylated peptides was achieved from 500 μg of IMAC-purified protein digest before 2D-LC-MS/MS analyses on a LTQ-Orbitrap Elite. 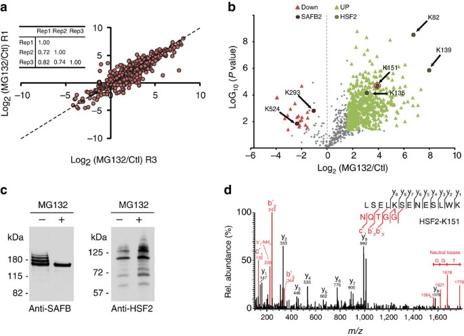Figure 3: Large-scale LC-MS/MS analysis of SUMOylated peptides following proteasome inhibition. (a) The correlation of the log2ratios for all quantified peptides after overnight treatment with 10 μM MG132 between two replicates is plotted (inset: correlation coefficients). (b) Volcano plot distribution of all 1042 SUMO peptides corresponding to 837 modified lysines on 469 proteins identified following MG132 treatment (false discovery rate: 2%). Green and red circles correspond to up and downregulated SUMOylated proteins, respectively. Arrows indicate sites for two selected proteins HSF2 and SAFB2. (c) Immunoblottings for SAFB2 and HSF2 showing differential SUMOylation after MG132 treatment. (d) MS/MS spectrum ofm/z674.00 from HSF2 with SUMOylated K151. SUMO3m remnant fragments ions (m/z132, 226, 243, 344) and the neutral losses (−NQ, −NQT, −NQTG, −NQTGG) are highlighted in red. Figure 3: Large-scale LC-MS/MS analysis of SUMOylated peptides following proteasome inhibition. ( a ) The correlation of the log 2 ratios for all quantified peptides after overnight treatment with 10 μM MG132 between two replicates is plotted (inset: correlation coefficients). ( b ) Volcano plot distribution of all 1042 SUMO peptides corresponding to 837 modified lysines on 469 proteins identified following MG132 treatment (false discovery rate: 2%). Green and red circles correspond to up and downregulated SUMOylated proteins, respectively. Arrows indicate sites for two selected proteins HSF2 and SAFB2. ( c ) Immunoblottings for SAFB2 and HSF2 showing differential SUMOylation after MG132 treatment. ( d ) MS/MS spectrum of m/z 674.00 from HSF2 with SUMOylated K151. SUMO3m remnant fragments ions ( m/z 132, 226, 243, 344) and the neutral losses (−NQ, −NQT, −NQTG, −NQTGG) are highlighted in red. Full size image The combined use of SUMO3m remnant immunoaffinity purification and label-free quantitative proteomics identified a total of 1215 SUMOylated peptides corresponding to 954 unique SUMOylation sites on 538 human proteins, of which 837 unique sites in 469 proteins were quantified ( Supplementary Data 1 ). A comparison of these data with those reported in Uniprot and Phosphositeplus databases indicated that 84% of identified proteins were not previously known to be SUMOylated, and that 86% of SUMO3m sites are novel. Although only 76 SUMO3m sites were previously reported, other sites were known to be ubiquitylated (303 sites) or acetylated (124 sites). Interestingly, we also identified 30 peptides modified by both SUMOylation and ubiquitylation, of which 20 peptides were only observed on proteasome inhibition. A large proportion of SUMOylated proteins were identified with one SUMO site, whereas 184 proteins contain two or more SUMO sites including hnRNP M that contained 15 SUMO sites ( Supplementary Data 1 ). The comparison of unique SUMOylated peptides showed a high correlation of fold-change ratio ( Fig. 3a ) with a limited number of peptides (<5%) detected in only one replicate ( Supplementary Fig. 6 ). We profiled changes in the abundance of SUMOylated peptides across replicates and determined that 61% of quantifiable peptides showed a threefold increase in SUMOylation on proteasome inhibition ( Fig. 3b ). The proportion of peptides that were unaffected or decreased in SUMOylation following MG132 treatment corresponded to only 37 and 2%, respectively. These experiments enabled the identification of SUMOylation sites in proteins previously known to be SUMOylated in response to proteasome inhibition including hnRNP M, PIAS1 and MCM7 (ref. 31 ). We performed separate immunoblot experiments on IMAC-enriched nuclear extracts ( Fig. 3c ) and confirmed the changes in SUMOylation of different endogenous substrates following MG132 treatment, such as scaffold attachment factor B2 (SAFB2) and heat-shock factor 2 (HSF2). These results are consistent with those obtained from label-free quantitative proteomics analyses where one of the three modified lysines of SAFB2 (K524) showed more than threefold decrease in SUMOylation in MG132-treated cells. We also identified four upregulated SUMOylation sites on HSF2 (K82, K135, K139 and K151), including K151, a site not previously known to be SUMOylated ( Fig. 3b ). The MS/MS spectrum of the corresponding peptide ( Fig. 3d ) showed backbone sequence ions together with characteristic SUMO remnant fragment ions and neutral losses that confirmed the sequence assignment and the modified K151 residue. We next analysed the distribution of all 20 amino acids for their propensity to be found proximal to SUMOylated lysines. We generated a heat map that represents the frequency of each residue at any of the ten positions upstream and downstream of the modified lysines, and compared this distribution with that observed for lysines of the human proteome ( Supplementary Fig. 7 ). This analysis confirmed the enrichment of aspartate and glutamate at the +2 position and of aliphatic residues at the −1 position, consistent with the canonical SUMO consensus sequence. This motif represented 49% of identified SUMOylation sites and showed a 4.5-fold enrichment compared with lysines from the human proteome. Consistent with previous reports, we also identified a reverse SUMO consensus motif [22] that represented 18% of all identified sites, whereas 33% of sites did not fall into any of the previously known motifs ( Fig. 4a ). 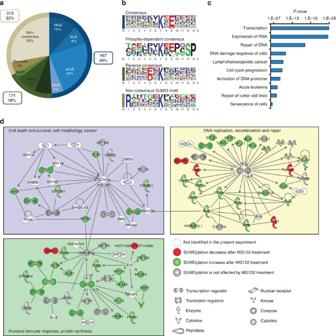Figure 4: Bioinformatic analysis of SUMOylated proteins and SUMO-modified lysines. (a) Pie chart distribution of the identified SUMO3m sites based on sequence motif. SUMO3m sites located within a SUMO consensus sequence are represented in blue, SUMO reverse consensus sequence are represented in green and SUMO sites located at non-consensus SUMO sequences are shown in grey. (b) Motif-X analysis of the SUMO sites identified in this study. The penultimate serine residue of the phospho-dependent consensus is phosphorylated. (c) Distribution of all the identified proteins based on their functional terms according to Ingenuity Pathway Analysis. (d) Subnetwork representation of SUMOylated proteins associated with cell survival, DNA replication and DNA repair, and protein synthesis. Figure 4: Bioinformatic analysis of SUMOylated proteins and SUMO-modified lysines. ( a ) Pie chart distribution of the identified SUMO3m sites based on sequence motif. SUMO3m sites located within a SUMO consensus sequence are represented in blue, SUMO reverse consensus sequence are represented in green and SUMO sites located at non-consensus SUMO sequences are shown in grey. ( b ) Motif-X analysis of the SUMO sites identified in this study. The penultimate serine residue of the phospho-dependent consensus is phosphorylated. ( c ) Distribution of all the identified proteins based on their functional terms according to Ingenuity Pathway Analysis. ( d ) Subnetwork representation of SUMOylated proteins associated with cell survival, DNA replication and DNA repair, and protein synthesis. Full size image Separate analyses of our SUMOylation data using Motif-X [32] identified four main SUMO motif categories with variation of flanking residues ( Fig. 4b ). For example, we identified the SUMO consensus motif with C-terminal clusters of acidic residues (negatively charged amino acid-dependent SUMOylation motif) [33] and a phospho-dependent SUMOylation motif [34] . In addition to the reverse SUMO consensus sequence, Motif-X analyses revealed an unsuspected RTHTGEKP motif in 49 sites (44 proteins), of which 17 sites (15 proteins) are localized on zinc finger proteins. SUMOylation targets included several cyclin-dependent kinases (for example, CDK1, CDK4 and CDK11b), transcription factors (for example, ATF2, ATF4, MAF and MYC) and disease-related proteins, such as promyelocytic leukemia (PML), parafibromin (CDC73), breast cancer type 1 susceptibility protein, Bloom syndrome protein. Gene Ontology terms analyses revealed a significant enrichment in functional groups associated with transcription ( P -value: 1.24E−25, Fisher’s exact test), expression of RNA ( P -value: 2.38E−25), DNA repair ( P -value: 6.42E−18) and cell cycle progression ( P -value: 1.59E−10) ( Fig. 4c ). We identified that histone H2A, H2B, H3 and H4 isoforms are SUMOylated, as are histone deubiquitinase (MYSM1), histidine methyltransferases (EHMT1 and SETDB1), histone acetyltransferase (KAT7) and subunits of histone deacetylases (SAP18, SAP130 and HDAC1), suggesting that SUMOylation contributes to epigenetic gene regulation and DNA repair through multiple pathways. Many SUMOylated substrates are involved in proteasome degradation pathways such as ubiquitin-activating enzymes, ubiquitin ligases and 26S proteasome regulatory subunits, supporting the notion that SUMO conjugation and the ubiquitin–proteasome system act in a cooperative manner [31] . Similar to other studies, we identified SUMO–SUMO branched conjugates and mixed SUMO-ubiquitin chains with the SUMOylation of ubiquitin (K11, K48 and K63) and the ubiquitylation of SUMO3 (K7) [35] . We used our SUMOylation data to generate a protein interaction network using Ingenuity Pathway Analysis that integrates known and predicted interactions from different sources. We combined interactions found in human and mammalian orthologues, resulting in a network of 301 proteins (nodes) and 2,465 connections (edges). This interaction network together with protein annotations highlighted different subsets of proteins associated with DNA replication and repair, cell death and survival, and protein synthesis ( Fig. 4d ). CDC73 SUMOylation affects its nucleocytoplasmic localization To further validate the identification of SUMOylated substrates and understand the biological significance of this modification on protein function, we selected the tumour suppressor CDC73 for subsequent in vitro SUMOylation assays and site-directed mutagenesis experiments. This protein is a member of the polymerase-associated factor 1 complex that plays important roles in the recruitment and activation of enzymes that modify histones, transcriptional elongation and the association of cleavage and polyadenylation factors with RNA Pol II [29] . Importantly, CDC73 is known to act as a tumour suppressor that inhibits cyclin D1 and c-Myc by recruiting the SUV39H1 histone methyltransferase, but can have tumour-promoting functions by binding to β-catenin, to induce the expression of Wnt target genes [36] . Label-free quantitative proteomics analysis of HEK293 cells expressing SUMO3m identified CDC73 as an upregulated SUMOylation target following proteasome inhibition. Our study identified five SUMOylation sites on CDC73 (K136, K161, K198, K283 and K301), a protein that until very recently was not known to be SUMOylated. Indeed, a report published during the review of this manuscript identified K136, K301 and K385 as SUMOylated residues on CDC73 (ref. 37 ). It is noteworthy that a recent large-scale proteomics study performed on MG132-treated Jurkat cells identified 12 ubiquitylation sites on CDC73, of which 4 sites were identified in our study (K136, K161, K198 and K283) [38] . However, all ubiquitylated sites identified on CDC73 remained either unchanged or showed a decrease in ubiquitylation on MG132 treatment. Two of the sites (K283 and K301) identified in our study are located in the C-terminal domain that interacts with RNA Pol II and one site (K136) is situated within the nuclear localization sequence (NLS) ( Fig. 5a ). To confirm that CDC73 is a direct substrate of Ubc9 and validate the position of the modified residues, we purified the recombinant His 6 -CDC73 from Escherichia coli for in vitro SUMOylation assays. Proteins from these assays were digested with trypsin and subjected to LC-MS/MS analyses as described before. These experiments confirmed that four of the five sites identified on CDC73 in vivo (K136, K161, K198 and K283) were directly SUMOylated by recombinant Ubc9 in vitro ( Supplementary Fig. 8 ). 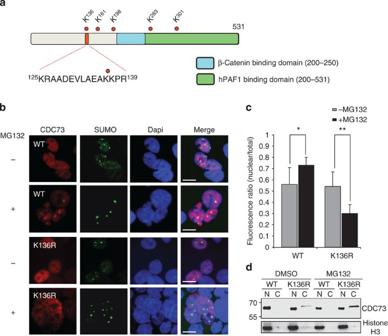Figure 5: SUMOylation of CDC73 at K136 affects its nucleocytoplasmic localization. (a) Distribution of SUMOylation sites identified on CDC73. Four SUMO sites (K136, K161, K198 and K283) were confirmed byin vitroSUMOylation assay. K198 and K301 are located in a SUMO consensus sequence, K136 is in a reverse SUMO consensus sequence, while other identified sites showed non-consensus sequences. (b) Cells co-transfected with His-SUMO3 and Myc-CDC73 WT or Myc-CDC73 K136R were treated or not with MG132 and double immunofluorescence were performed with anti-Myc and anti-His antibodies (scale bar, 10 μm). (c) Intracellular distribution of fluorescent signal for CDC73 WT and CDC73 K136R mutant for control and MG132-treated cells. The graph shows the ratio of the nuclear signal compared with the total cell signal (*P=0.01, **P=0.0001, Student’st-test,n=10 cells per condition). (d) Immunoblottings against CDC73 for nuclear and cytoplasmic extracts obtained for control (DMSO) and MG132-treated HEK293 cells expressing CDC73 WT or CDC73 K136R. The immunoblots indicate that CDC73 K136R is partially translocated to the cytoplasm under proteasome inhibition. Control loading for nuclear extract is shown for histone H3. Figure 5: SUMOylation of CDC73 at K136 affects its nucleocytoplasmic localization. ( a ) Distribution of SUMOylation sites identified on CDC73. Four SUMO sites (K136, K161, K198 and K283) were confirmed by in vitro SUMOylation assay. K198 and K301 are located in a SUMO consensus sequence, K136 is in a reverse SUMO consensus sequence, while other identified sites showed non-consensus sequences. ( b ) Cells co-transfected with His-SUMO3 and Myc-CDC73 WT or Myc-CDC73 K136R were treated or not with MG132 and double immunofluorescence were performed with anti-Myc and anti-His antibodies (scale bar, 10 μm). ( c ) Intracellular distribution of fluorescent signal for CDC73 WT and CDC73 K136R mutant for control and MG132-treated cells. The graph shows the ratio of the nuclear signal compared with the total cell signal (* P =0.01, ** P =0.0001, Student’s t -test, n =10 cells per condition). ( d ) Immunoblottings against CDC73 for nuclear and cytoplasmic extracts obtained for control (DMSO) and MG132-treated HEK293 cells expressing CDC73 WT or CDC73 K136R. The immunoblots indicate that CDC73 K136R is partially translocated to the cytoplasm under proteasome inhibition. Control loading for nuclear extract is shown for histone H3. Full size image The CDC73 SUMOylation sites are located in different structural domains and could therefore affect several distinct functions of CDC73. We surmised that attachment of SUMO to sites proximal to the NLS could affect the nuclear localization of CDC73, consistent with accumulating evidences on the interplay between nuclear transport and ubiquitin/SUMO modifications [39] . To test this hypothesis, HEK293 cells co-transfected with constructs expressing His-SUMO3 and Myc-CDC73 WT or Myc-CDC73 SUMOylation site mutants were treated or not with MG132, and immunofluorescence experiments were performed to monitor Myc-CDC73 and SUMO3 localization. These experiments indicated that a portion of CDC73 WT proteins form dense nuclear speckles on proteasome inhibition that co-localize with SUMO3 within PML nuclear bodies (NBs) ( Fig. 5b and Supplementary Fig. 9 ). To evaluate the functional significance of SUMOylation at individual sites, we mutated lysine K136, K161, K198 or K283 to arginine and monitored the nuclear localization of Myc-CDC73 mutants by immunofluorescence ( Fig. 5c and Supplementary Fig. 10 ). These experiments revealed that K136 was the only site that affected the nucleocytoplasmic localization of CDC73 ( Fig. 5b and Supplementary Fig. 10 ). Although Myc-CDC73 localized specifically in the nucleus, Myc-CDC73 K136R mutant was partially translocated to the cytoplasm and no longer localized in PML NBs on MG132-treatment ( Fig. 5c and Supplementary Fig. 10 ). Immunoblot analyses of nuclear and cytoplasmic extracts from cells co-transfected with His-SUMO3 and Myc-CDC73 WT or Myc-CDC73K136R confirmed that Myc-CDC73 WT was found in the nucleus while Myc-CDC73 K136R was partially translocated to the cytosol following proteasome inhibition ( Fig. 5d ). The independent confirmation of SUMOylation of K136 by Tammsalu et al. [37] , in addition to the absence of changes in the ubiquitylation of CDC73 K136 on MG132 treatment, support a role for SUMOylation in the nuclear retention of CDC73. This finding is consistent with a recent study on the E1 SUMO-activating enzyme SAE2, indicating that SUMOylation of several residues located within the NLS and adjacent to the NLS regions was required for the nuclear retention of SAE2, whereas the non-SUMOylatable form of SAE2 was rapidly exported to the cytoplasm [40] . Altogether, our data suggest that SUMOylation of CDC73 at K136 is required for its retention in the nucleus and its localization within PML NBs, thus providing novel insights on potential roles of SUMOylation in the regulation and nucleocytoplasmic retention of CDC73. The use of a highly selective antibody recognizing SUMO remnants facilitated the global analysis of human SUMO proteome and enabled the identification of ~950 sites in ~500 proteins. Approximately half of the identified sites were represented by the canonical SUMO consensus sequence (ψK x E) recognized by Ubc9, whereas ~20% of the sites corresponded to a reverse consensus motif. Detailed analysis of the remaining sites revealed an unexpected motif defined by RTHTGEKP that was mostly encountered between C2H2 tandem repeats of zinc finger proteins. We also noted that several SUMOylated proteins known to bind DNA and RNA also contained an arginine residue at position −6 from the SUMOylated lysine including pre-mRNA-splicing factor SLU7 (K199 and K408), splicing factor U2AF (K125), non-POU domain-containing octamer-binding protein (K371) and DNA replication licensing factor MCM7 (K159). These observations raise the possibility that SUMOylation plays a role in the dynamic regulation of DNA and RNA protein interactions. Further studies are needed to examine whether the SUMOylation of zinc finger proteins occurs under truly physiological conditions and to determine the signalling mechanism leading to this modification. SUMO remnant immunoaffinity purification was combined with label-free quantitative proteomics to monitor changes in protein SUMOylation in response to proteasome inhibition. The ubiquitin–proteasome system is an important component of cellular SUMO2/3 cycle required for the processing of SUMO targets and for the recycling of SUMO2/3. Previous reports described a cross-talk between ubiquitylated and SUMO-modified proteins in PML NBs leading to an accumulation of ubiquitin-associated SUMO2/3 conjugates under proteosomal inhibition [9] , [31] , [41] . Consistent with these findings, we determined that a large proportion of SUMO sites (61%) identified in HEK293 cells stably expressing SUMO3m showed a threefold increase in SUMOylation on MG132 treatment. Interestingly, 2% of regulated sites from different proteins showed a decrease in SUMOylation including histones, SAFB2, 60S ribosomal proteins L26, and remodelling and spacing factor 1. Removal of SUMO3m from abundant SUMOylated proteins such as histones H2B and H3 might be necessary to compensate for the depleted pool of free SUMO3m, a situation previously observed for ubiquitin during proteasome inhibition [42] . Our results demonstrate that the use of antibodies recognizing SUMO remnants can be applied to the isolation of SUMO acceptor lysines present at low abundance in protein extracts of human cells. This approach opens up new avenues to identify protein substrates, their paralogue-specific SUMOylation sites, the interplay with protein ubiquitylation and the regulation of protein SUMOylation on different environmental conditions. Materials Modified porcine sequencing grade-modified Trypsin was obtained from Promega (Madison, WI, USA). Acetonitrile was purchased from Fisher Scientific (Whitby, ON, Canada). Ammonium bicarbonate and formic acid were obtained from EM Science (Mississauga, ON, Canada). Ammonium hydroxide, trifluoroacetic acid, DTT (DL-dithiolthreitol), chloroacetamide, protease inhibitor cocktail (4-(2-aminoethyl)benzenesulfonyl fluoride, pepstatinA, E-64, bestatin, leupeptin and aprotinin), phosphatase inhibitor cocktail (sodium vanadate, sodium molybdate, sodium tartrate and imidazole) serum-free were purchased from Sigma-Aldrich (Oakville, ON, Canada). Bradford protein assays were obtained from Bio-Rad (Mississauga, ON, Canada). Tris was purchased from EMD Omnipur (Lawrence, KS). Bond breaker TCEP (Tris[2-carboxyethyl] phosphine) was purchased from Pierce Biotechnology Inc. (Rockford, IL). PBS and EDTA were obtained from HyClone (Thermo Scientific, Logan, UT). Oasis HLB cartridges (1 cc, 30 mg) were purchased from Waters (Milford, MA). ECL chemiluminescence detection system was purchased from Amersham Pharmacia Biotech (Montréal, QC, Canada). Antibodies anti-SAFBII (Ab8060) and anti-HSF2 (Ab52758) were purchased from Abcam (Toronto, Canada). Mouse anti-PML (sc-966) and rabbit anti-α-Myc (9E10, sc-789) were obtained from Santa Cruz, and mouse anti-His (penta-His, 34660) was from Qiagen. Goat anti-mouse IgG and goat anti-rabbit IgG secondary antibodies were purchased from Millipore (Ottawa, ON, Canada). Solvents for chromatographic analysis were all HPLC grade (Fisher Scientific and in-house Milli-Q water). Capillary HPLC columns for nano-LC-MS were packed in-house using Jupiter C18 (3 μm) particles from Phenomenex (Torrance, CA) and fused silica tubing from Polymicro Technologies (Phoenix, AZ). All tryptic peptides with SUMO remnant chains were synthesized by automated SPOT synthesis as described previously [30] . Generation of hybridoma cells Hybridoma clones were produced by Epitomics (Burlingame, CA) from immunized rabbits. Briefly, peptides (F{K(GGTQE)}GEC) and (F{K(GGTQN)}GEC) were conjugated with keyhole limpet haemocyanin as immunogens and two rabbits were immunized using standard immunization of three injections. Preliminary binding assays were performed on test bleeds (5 ml each) from each rabbit. Splenectomy was conducted on one rabbit 4–8 weeks post injection boost to isolate lymphocytes from the spleen and perform hybridoma fusion. An enzyme-linked immunosorbent assay screen was performed against the immunizing antigens conjugated to BSA and positive clones were expanded in 24-well plates. Hybridomas clones UMO 1 were selected after confirmation of their affinity by enzyme-linked immunosorbent assays conducted against unconjugated antigens. Cells of monoclonal clones were grown in MegaCell DMEM (pH 7.2, Sigma) supplemented with 10% fetal bovine serum, 50 μg ml −1 of kanamycin, 1 mM glutamine, and cells were split and cell culture supernatant was collected every week. Hybridoma clones UMO1 were isolated in 48 different plates. Antibodies from these clones were used for immunoprecipitation of synthetic SUMO remnant-containing peptides spiked in tryptic digests of WT HEK293 cells to assess the degeneracy of antibodies. Clone UMO 1–7 provided the highest recoveries of synthetic SUMO remnant-containing peptides (DAAVSK*K, EFK*EVLK, TVIK*KEEK, VIK*MESEEGK, TDGFDEFK*VR and LLVHMGLLK*SEDK, where * indicates the modified lysine residues). A set of ten subclones was generated from UMO 1–7 hybridoma clone and further screened using synthetic SUMO remnant-containing peptides. The clone UMO 1-7-7 provided the highest recoveries of synthetic peptides and was selected for subsequent experiments. The monoclonal antibody from UMO 1-7-7 clone was purified by Protein A affinity column and was found to bind peptides containing modified lysines with any of the SUMO remnant chain in a wide range of sequence contexts ( Supplementary Figs 1 and 2 ). The UMO 1-7-7 anti-SUMO remnant–lysine monoclonal antibody was found to be IgG1 isotype. Cell culture HEK293 obtained from ATCC were transformed to stably express SUMOm by transfecting cells with pcDNA SUMO constructs and subsequent neomycine selection as described previously [11] . HEK293 stably expressing 6xHis-SUMO-3-Q87R-Q88N cells (SUMO3m) were maintained in DMEM medium (HyClone, Ontario, Canada) containing 10% fetal bovine serum, 1% L -glutamine, 1% penicillin/streptomycin, neomycine (0.5 mg ml −1 ) and cultured at 37 °C in a 5% CO 2 constant atmosphere. For western blotting, immunofluorescence studies and MS analyses, cells were treated with 10 μM of MG132 (Z-Leu-Leu-Leu-al, M7449, Sigma-Aldrich, St Louis, MO) during 16 h. Cell fractionation and enrichment of SUMOylated proteins HEK293 cells (5 × 10 8 cells per replicate) stably expressing 6xHis-SUMO-3-Q87R-Q88N were grown as described previously [11] and treated using 10 μM MG132 for 8 h. After treatment, cells were rinsed using PBS, lysed in hypotonic buffer (10 mM Tris-HCl, pH 7.65, 1.5 mM MgCl2, 1 mM DTT, 20 mM N-ethylmaleimide and proteases inhibitors) and centrifuged at 215 g . The supernatant constituted the cytoplasmic fraction. The nuclear pellet was resuspended in buffer A (6 M guanidinium HCl, 0.1 M NaH2PO4, 0.01 M Tris-HCl, pH 8, 10 mM β-mercaptoethanol), sonicated, centrifuged at 16,000 g and added to 500 μl of Ni-NTA beads for 3 h at room temperature. The total protein amount was quantitated by Bradford protein assay. Beads were then centrifuged and wash once with 1 ml of buffer A, five times with 1 ml of buffer B (8 M urea, 0.1 M NaH 2 PO 4 , 0.01 M Tris–HCl, pH 8, 10 mM β-mercaptoethanol, 0.02 mM imidazole). Trypsin digestion was realized directly by suspending beads in 8 M urea. Proteins were reduced in 5 mM TCEP for 20 min at 37 °C and then alkylated in 5 mM chloroacetamide for 20 min at 37 °C. A solution of 5 mM DTT was added to the protein solution to react with the excess chloroacetamide. Samples were diluted to 1 M urea and proteins were digested in 50 mM ammonium bicarbonate with modified trypsin overnight (1:50 enzyme:substrate ratio) at 37 °C under high agitation speed. The digest was acidified with trifluoroacetic acid, desalted using an HLB cartridge (Waters) and then dried down by Speed Vac. Samples were resuspended in 200 μl of a solution (100 mM Tris, 150 mM NaCl). The immuno-affinity purification was then realized on peptide using the antibody to a final ratio of 3:1 (antibody:protein) and incubated overnight at 4 °C. The samples were then transferred onto a microcon cutoff 30 kDa (NanoSep Pall), centrifuged, wash three times with 300 μl of tris buffer saline, TBS 1 × (20 mM Tris, 150 mM NaCl), washed two times with 300 μl of TBS 0.1 × and once with water for a complete desalting of the sample. Peptide elution was performed four times using 100 μl with a solution of 0.2% formic acid and then dried down by Speed Vac prior to MS analyses. Immunoblot analysis The lysates were boiled 5 min in Laemmli buffer (10% (w/v) glycerol, 2% SDS, 10% (v/v) 2-mercaptoethanol and 0.0625 M Tris–HCl, pH 6.8) and separated by SDS–PAGE followed by electroblotting onto nitrocellulose membrane. After blocking of nonspecific binding sites with 5% non-fat milk, the membranes were incubated with primary antibody (SUMO1, SUMO2/3, SAFB2, HSF2, Histone H3 or α-Myc) followed by horseradish peroxidase-conjugated secondary antibody. The secondary antibody was detected with the ECL chemiluminescence detection system. Uncropped scans of the most important immunoblots are included in Supplementary Fig. 11 . Plasmid constructs and site-directed mutagenesis Total cellular RNA from human cell (HEK293 WT) was extracted using TRIzol Reagent (Invitrogen) according to the manufacturer’s instructions. Two micrograms of total ARN was used to synthesize the complementary DNA using Omniscript reverse transcriptase (Qiagen) in a volume of 20 μl. Two microlitres of this cDNA was subsequently used for PCR analysis. The pcDNA3-Myc-HsCDC73-WT expressing Myc-tagged CDC73 were realized using the complete CDC73 human coding sequence amplified with CDC73 forward primer: 5′-CACTTGAATTCATGGCGGACGTGCTTAGCG-3′; CDC73 reverse primer: 5′-CACTTCTCGAGTCAGAATCTCAAGTGCGATTTATGC-3′. PCR products were digested with EcoRI and XhoI, gel purified and individually inserted into pcDNA3-N-Myc vector (gift from Dr Sébastien Michaud, Université Laval) at the corresponding site previously treated with the same restriction enzymes to generate fusion protein bearing an N terminus Myc tag. Mutagenesis was carried out by PCR. The mutations were made in the plasmid template pcDNA3-N-Myc-HsCDC73-WT using the GeneART Site-Directed Mutagenesis System (Invitrogen Life Technology, Carlsbad, CA) according to the manufacturer’s protocol. Base substitution mutagenic oligonucleotide overlapping primers corresponding to position single mutants were performed for HsCDC73 on K136R, K161R, K198R and K283R. All plasmids were verified by sequencing. Cell transfection HEK293 cells were plated 20 h in advance at a desired confluence. Cells were washed once with the culture medium and incubated 24 h in medium containing the plasmid:Fugene HD (Roche Diagnostics Canada, Laval, QC) complex (ratio 2 μg DNA:9 μl Fugene HD) prepared according to the manufacturer’s protocol. All plasmids pcDNA3-Myc-HsCDC73 or CDC73 SUMO-deficient mutants were co-transfected with a plasmid expressing SUMO3 WT. After incubation, the medium was changed and left another 24 h before subsequent experiments. Immunofluorescence analysis Cells were growth on cover slips and transfected as described previously. After treatment, cells were washed with PBS (three times), fixed using 4% paraformaldehyde for 10 min and rinsed with PBS. Cells were then permeabilized (PBS, 0.2% Triton) for 5 min, rinsed in PBS, saturated (PBS 5% BSA, 0.1% tween) for 30 min and washed again. Cells were incubated for 2 h with the first antibody (α-Myc and His or Myc and PML), rinsed and incubated for 45 min with the corresponding Alexafluor antibody combination (AlexaFluor 488 and AlexaFluor 594, Invitrogen). Cells were washed and stained with 4',6-diamidino-2-phenylindole and washed again. Cover glasses were fixed on slide using Mowoil mounting media. Immunofluorescence images were acquired on a Nikon Eclipse TE2000-E inverted confocal laser scanning microscope using an Apochromat × 100 oil-immersion objective. Mass spectrometry LC-MS/MS analyses were performed on a nano-LC 2D pump (Eksigent) coupled to an LTQ-Orbitrap Elite hybrid mass spectrometer via a nanoelectrospray ion source (Thermo Fisher Scientific). The peptide mixture was separated on an SCX trap column, 5 μm, 300 Å, 0.5 ID × 23 mm (Optimize Technologies) before elution on line to a 360-μm ID × 4 mm, C18 trap column and separated on a 150 μm ID × 15 cm nano-LC column (Jupiter C18, 3 μm, 300 Å, Phenomex). The SCX separation was performed using salt pulses of 0, 250, 500, 750, 1,000 and 2,000 mM ammonium acetate, pH 3.5. The peptide separation was performed using a linear gradient from 5% to 40% (aqueous acetonitrile, 0.2% formic acid) in 53 min at 600 nl min −1 . Survey scan were acquired after accumulation of 10 6 ions in the linear ion trap for m/z 300–2,000 using a resolution of 60,000 at m/z 400. Mass calibration used a lock mass from ambient air (protonated (Si(CH 3 ) 2 O)) 6 ; m/z 445.120029) and provided mass accuracy within 8 p.p.m. for precursor ion mass measurements. The six most intense precursor ions from the survey scan were selected for fragmentation in the HCD cell. Precursor ions were accumulated for a maximum of 300 ms to reach a target value of 50,000. Fragment ions were obtained in the HCD collision cell at normalized collision energy of 30% before their transfer to the Orbitrap analyser operating at a resolution of 30,000 at m/z 400. The dynamic exclusion of previously acquired precursor ions was enabled (repeat count 1, repeat duration: 30 s; exclusion duration: 45 s). Peptide and protein identification Peak lists were generated using Mascot distiller (version 2.3.2.0, Matrix Science) and MS/MS spectra were searched against a concatenated forward/reverse Uniprot Swiss-Prot Human, containing 37,265 forward sequences (released 4 February 2013) using Mascot (version 2.3.2, Matrix Science) to achieve a false discovery rate of <2%. MS/MS spectra were searched with a mass tolerance of 8 p.p.m. for precursor ions and 0.02 Da for HCD spectra. The number of allowed missed cleavage sites for trypsin was set to 2 and phosphorylation (STY), oxidation (M), deamidation (NQ), carbamidomethylation (C), ethylmaleimidation (C), ubiquitylation (K), acetylation (K, N term) and SUMOylation (NQTGG for SUMO3), (K) were selected as variable modifications. A software application was developed to search Mascot generic files (mgf) for specific SUMO3 fragment ions ( m/z 132.0768, 226.0822, 243.1088, 326.1459, 327.1299, 344.1565, 383.1674, 401.1779 and 458.1994, and neutral losses of SUMO remnants) to produce a subset mgf file containing only MS/MS spectra of potential SUMOylated peptide candidates. SUMO fragment ions were removed from the mgf files and each MS/MS spectrum was searched for fragment ions corresponding to cleavage of the SUMO remnant chain (consecutive losses of a T, TG and TGG). Fragment ions corresponding to the branched SUMO chain were removed from the MS/MS spectra before conducting the database search with Mascot. Manual inspection of all MS/MS spectra for modified peptides was performed to validate assignments. The software enabling the selection and removal of SUMO fragment ions is available at http://proteomics.iric.ca/tools/MSMSEditor/ . For label-free quantitative proteomics analyses, Orbitrap raw LC-MS data files were transformed into peptide maps using in-house peptide detection and clustering software [43] . Peptide maps belonging to one experiment were clustered and aligned using clustering parameters of Δ m/z : 0.02 and time tolerance of ±2 min (wide), ±0.5 min (narrow). For each LC-MS run, we normalized peptide ratios so that the median of their logarithms was zero, to account for unequal protein amounts across conditions and replicates. Intensities were summed across SCX fractions for peptides of identical sequences. Peptide clusters were aligned with mascot identification files to assign sequence identity. Bioinformatic analyses The density map for the SUMOm-remnant-modified lysines was calculated by taking a subset of protein sequence, ten amino acids on either side of modified lysines from the whole protein sequence. The frequency of each of the 20 individual amino acids at each position from −10 to +10 was calculated for modified lysines and this value was normalized to the frequency of the same amino acid at the same position using all lysines in the human Swiss-Prot database (released February 2013) to obtain a relative ratio. The highest relative ratio detected was 4.5 and the range of the colour map was set accordingly. Enrichment and depletion of amino acids were determined following a Fisher’s exact test. The analysis of regulatory interaction network in the human system was performed using Ingenuity Pathways Analysis (Ingenuity Systems). A data set containing protein identifiers (Uniprot Ids) was uploaded into in the application. Each protein identifier was mapped to its corresponding gene object in the Ingenuity Pathways Knowledge Base. Genes or gene products are represented as nodes, and the biological relationship between two nodes is represented as an edge (line). All edges are supported by at least one reference from the literature or from canonical information stored in the Ingenuity Pathways Knowledge Base. The intensity of the node colour indicates the degree of up- (green) or down- (red) regulation in our filter array experiment. Nodes are displayed using various shapes that represent the functional class of the gene product. Edges are displayed as solid (direct interaction) or dashed (indirect interactions) lines with and without arrowheads. Various colours that describe the nature of the relationship between the nodes were added manually in Adobe Illustrator. The functional analysis of a network identified the biological functions that were most significant to the genes in the network (Fisher’s exact test). Accession Codes . The proteomic data associated with this manuscript has been uploaded to Peptide Atlas ( http://www.peptideatlas.org ) under accession code PASS00461. How to cite this article: Lamoliatte, F. et al. Large-scale analysis of lysine SUMOylation by SUMO remnant immunoaffinity profiling. Nat. Commun. 5:5409 doi: 10.1038/ncomms6409 (2014).